Telomerase reverse transcriptase promoter mutations in primary cutaneous melanoma We previously reported a disease segregating causal germline mutation in a melanoma family and recurrent somatic mutations in metastasized tumours from unrelated patients in the core promoter region of the telomerase reverse transcriptase ( TERT ) gene. Here we show that the TERT promoter mutations, besides causing an increased gene expression, associate with increased patient age, increased Breslow thickness and tumour ulceration in 287 primary melanomas. The mutations are more frequent at both intermittently and chronically sun-exposed sites than non-exposed sites and tend to co-occur with BRAF and CDKN2A alterations. The association with parameters generally connected with poor outcome, coupled with high recurrence and mechanistic relevance, raises the possibility of the eventual use of TERT promoter mutations in the disease management. Cutaneous melanoma, one of the most aggressive form of skin cancers owing to its high propensity to metastasize and intrinsic drug resistance, accounts for the majority of skin-cancer-related deaths [1] . Sun exposure coupled with characteristic phenotypes define the most important risk factors for developing melanoma [2] . Sequencing data have shown that of all cancer types, melanoma genomes are marked by the highest prevalence of somatic mutations and mutational pattern depict a characteristic ‘ultraviolet-signature’, indicated by a high rate of transitions at dipyrimidinic sites [3] , [4] , [5] . Frequently mutated genes are involved in various signalling cascades and cell cycle regulation. Besides the recurrent alterations in BRAF / NRAS , CDKN2A , PTEN and others, various sequencing projects have also identified mutations in a number of additional genes including GRIN2A , RAC1 , BCL2L12 , PPP6C and STK19 (refs 4 , 5 , 6 , 7 , 8 ). We previously described a highly penetrant, disease segregating causal germline mutation in a melanoma family and recurrent somatic mutations in tumours from unrelated patients within the core promoter region of the telomerase reverse transcriptase ( TERT ) gene [9] . The somatic mutations in the TERT promoter simultaneously discovered in another study have been shown to be frequent in a wide range of cancer types [10] , [11] , [12] , [13] , [14] , [15] . The familial germline A>C mutation at −57 bp (from ATG start site; Chr 5:1,295,161 hg19 co-ordinate) and the recurrent mutually exclusive C>T somatic mutations at −124 (1,295,228) bp and −146 (1,295,250) bp resulted in creation of E-twenty six/ternary complex factor (Ets/TCF)-binding motifs with consequent tumour-specific increased TERT expression as shown by gene reporter assays [9] , [10] . The frequency of the alterations in the TERT promoter exceeded that of any known gene mutation in melanoma. The widespread occurrence of the TERT promoter mutations in many cancers has now been confirmed. The mutations have been associated with an increased gene expression, decreased telomere length and adverse forms of the disease and poor outcome [11] , [16] , [17] , [18] , [19] , [20] , [21] . Here we screen 287 primary cutaneous melanomas to validate the presence of mutations in primary melanoma and to find association, if any, with different parameters. We analyse the data for association with different phenotypic, epidemiologic and clinical features. The results show that activating TERT promoter mutations, which result in an increased gene expression, associate with increased Breslow thickness and tumour ulceration. The mutations are more frequent at sun-exposed than at non-exposed sites and tend to co-occur with BRAF and CDKN2A alterations. The findings, if confirmed, coupled with high recurrence and mechanistic relevance, raise the possibility of the eventual use of TERT promoter mutations in disease management. Tumour information and sequencing In this study we screened primary tumours from 287 melanoma patients. Of 287 tumours, 227 were formalin-fixed paraffin-embedded (FFPE) tumour tissues for which corresponding mutational data for the BRAF and NRAS genes were available. Additional 60 tumours were available as fresh frozen tissues, which were, besides TERT promoter mutations, also sequenced for BRAF and NRAS . In addition, in those tumours alterations at the CDKN2A locus were determined using methylation-sensitive multiplex ligation-dependent probe amplification (MS-MLPA). 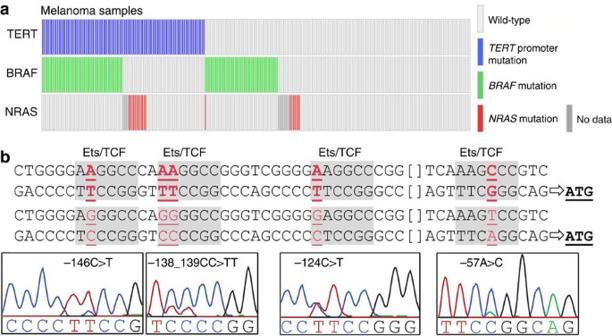Figure 1: Distribution of mutations in primary melanomas and representative sequences showing somatic mutations in theTERTpromoter. (a) The distribution of mutations in theTERTpromoter,BRAFandNRASgenes in 287 melanomas are indicated by different colours. (b) Representative sequences of theTERTpromoter from different tumours with mutations; −146C>T mutation shown in the left most panel followed by the −138/−139CC>TT tandem mutation, −124C>T and −57A>C. The wild-type and mutated sequences are shown on the top, and the Ets/TCF consensus motifs created by the mutations are marked. Detailed epidemiological data, phenotype information about the patients and the available tumour characteristics were available and are given in Supplementary Table 1 and Supplementary Data 1 . Mutations in the TERT promoter Mutations in the TERT promoter region were detected in 109 of 287 (37.9%) melanomas ( Table 1 ). The two mutually exclusive somatic changes −124C>T and −146C>T accounted for 91 of 109 (83.5%) mutations with the most common being the −146C>T (51 of 109; 46.8%). The position at −124 bp was altered in 36.7% (40/109) of tumours by the C>T transitions and one tumour carried a C>A transversion. Four tumours (3.7%) carried CC>TT tandem mutation at −124/−125 bp and seven tumours (6.4%) had a similar tandem mutation at the positions −138/−139 bp. A previously described causal A>C alteration at −57 bp in a melanoma family was present as a somatic mutation in 3 of 109 (2.8%) tumours with mutations ( Fig. 1 ). In addition, three tumours with the −146C>T mutation also carried a C>T base change at −149 bp position. One tumour with the −124C>T and another with the −138/−139CC>TT mutations also carried the −101C>T alteration. In total 15 tumours with mutations at −146, −124 and −138/−139 bp also carried additional alterations ( Table 1 ). In addition, eight melanomas carried exclusive mutations at various other positions within the core TERT promoter, which included −46C>T, −58C>T, −144C>T, −154CT, −156C>T, −176C>T, −187C>T and −242C>T. The observed alterations lead to putative changes in transcription factor-binding sites including creation of a Ets/TCF-binding motif by −156C>T ( Table 1 ) [22] . From six patients, besides primary tumours, additionally, metastases were also available. Out of those, five metastases were from five patients, whereas from one patient two metastases were available. Sequencing showed that primary and corresponding metastatic (four locoregional cutaneous and one locoregional lymph node) tumours from five patients did not carry mutations in the TERT promoter. In contrast, all three tumours from one patient, one primary and two metastases, showed the −124C>T and additional −91C>T mutations. Within the primary tumour and one metastasis (locoregional cutaneous), the TERT promoter mutations were heterozygous; in the second metastasis (soft tissue from maxillary mucosa) both mutations were in the homozygous state indicating loss of the wild-type allele ( Supplementary Fig. 1 ). Table 1 Types of TERT promoter mutations in primary melanomas. Full size table Figure 1: Distribution of mutations in primary melanomas and representative sequences showing somatic mutations in the TERT promoter. ( a ) The distribution of mutations in the TERT promoter, BRAF and NRAS genes in 287 melanomas are indicated by different colours. ( b ) Representative sequences of the TERT promoter from different tumours with mutations; −146C>T mutation shown in the left most panel followed by the −138/−139CC>TT tandem mutation, −124C>T and −57A>C. The wild-type and mutated sequences are shown on the top, and the Ets/TCF consensus motifs created by the mutations are marked. Full size image TERT promoter mutations and tumour characteristics Data analysis ( Supplementary Table 1 ) showed that the TERT promoter mutations were more frequent in tumours from melanoma patients aged above 65 years than from patients with age 65 years or below (odds ratio (OR): 2.01; 95% confidence interval (CI): 1.22–3.32; P =0.006, χ 2 -test). Similarly, TERT promoter mutations were more frequent in melanomas located at sun-exposed parts of the body. The association was statistically significant for chronically exposed sites (OR: 2.74; 95% CI: 1.30–5.78; P =0.008, χ 2 -test) as well as for intermittently exposed sites (OR: 4.44; 95% CI: 1.70–11.5; P =0.002, χ 2 -test). Presence of solar lentigines at the site of melanoma also increased the odds of TERT promoter mutations within the lesion (OR: 1.84; 95% CI: 1.12–3.01; P =0.02, χ 2 -test), although the mutations were not associated with presence of solar lentigines in general. Other factors, such as a personal history of sunburns, sunburns at the site of melanoma or outdoor work did not influence the presence of TERT promoter mutations. Similarly, the mutations did not show any association with any characteristic patient phenotype like hair, skin or eye colour or status of the MC1R gene. We found that acral lentiginous melanoma had the lowest frequency of the TERT promoter mutations (1/24, 4.2%). Nodular melanoma (NM), in contrast, had the highest frequency (42/76, 55.3%) of the mutations with an OR of 2.80 (95% CI: 1.63–4.92, P =0.0002, χ 2 -test) for comparison with all other tumour types. Three of 13 (23%) lentigo maligna melanoma tumours carried TERT promoter mutations. Frequencies of TERT promoter mutations were higher in vertical growth phase tumours than those in radial growth phase (OR: 3.97, 95% CI: 1.60–9.94, P =0.003, χ 2 -test). We observed statistically significant association between the TERT promoter mutation frequency and increasing Breslow thickness ( Supplementary Table 1 ). Ulcerated tumours were also found more likely to carry TERT alterations than non-ulcerated tumours (OR: 2.20, 95% CI: 1.30–3.67, P =0.003, χ 2 -test). The lesions from patients with locoregional or distant disease at presentation carried more TERT promoter mutations than those with in situ or localized melanomas (OR: 1.90, 95% CI: 1.17–3.38, P =0.01, χ 2 -test). A family history of melanoma or a past personal history of non-melanoma skin cancer or any other non-cutaneous neoplasia did not affect the odds of carrying a TERT promoter mutation. 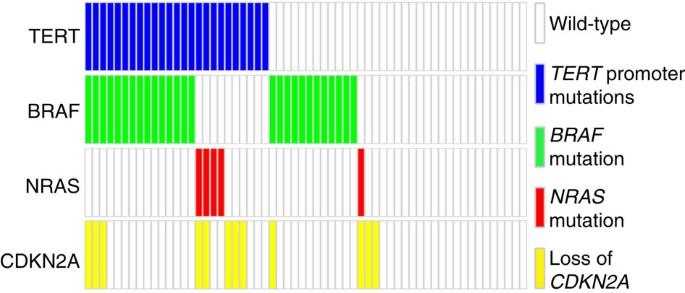Figure 2: Distribution of mutations in a subset of 60 primary melanomas. The distribution of mutations in theTERTpromoter,BRAFandNRASgenes and alterations inCDKN2Ain a subset of 60 fresh frozen melanoma tissues are indicated by different colours. In a multivariate model, we observed that the associations between TERT promoter mutations and histological subtypes, tumour stage and presence of solar lentigines were no longer statistically significant ( Table 2 ). The association between TERT promoter mutations and NMs was dependent on tumour ulceration and Breslow thickness, and not on patient’s age at diagnosis. Table 2 Multivariate analysis of TERT promoter mutations and various patient and tumour characteristics. Full size table TERT promoter mutations and alterations in other genes The BRAF mutations at codon 600 were present in 104 of 287 (36.2%) tumours and NRAS mutations were present in 20 of 275 (7.3%) melanomas. In 18 melanomas, mutations in NRAS affected codon 61, one melanoma carried a mutation in codon 13 and one melanoma carried a T58I mutation. The tumour affected by the latter mutation also harboured the V600E mutation in BRAF . Aberrations at the CDKN2A locus were detected in 12 of the 60 (22.2%) tumours ( Fig. 2 ). 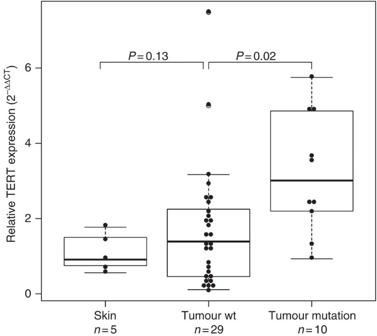Figure 3: RelativeTERTgene expressions in melanomas with and withoutTERTpromoter mutations. TERTmRNA expression measured by quantitative real-time PCR in skin tissues from healthy individuals (n=5), tumours without (n=29) and tumours with theTERTpromoter mutations (n=10). Expression ofTERTgene was normalized toGUSBexpression, used as an internal standard and quantification was done by ΔΔCTmethod with log2 transformation. Experiments were carried out in triplicate and box plots represent mean±s.e.m.Pvalues were determined byt-test. Four tumours carried mutations, seven had large deletions and the promoter specific for the p16 transcript was hypermethylated in two tumours ( Table 3 ). Figure 2: Distribution of mutations in a subset of 60 primary melanomas. The distribution of mutations in the TERT promoter, BRAF and NRAS genes and alterations in CDKN2A in a subset of 60 fresh frozen melanoma tissues are indicated by different colours. Full size image Table 3 Alterations in TERT promoter, 9p21 locus, BRAF and NRAS in a subset of melanomas*. Full size table Mutations in the TERT promoter were more frequent in tumours with BRAF mutations (OR: 2.50, 95% CI: 1.53–4.14, P =0.0003, χ 2 -test). A similar association between the TERT promoter mutations and NRAS mutations was observed (OR: 2.60, 95% CI: 1.03–6.62, P =0.04, χ 2 -test); however, it may be pointed out that data for NRAS mutations were available only for 274 tumours. In a subset of 60 melanomas, 12 tumours had CDKN2A aberrations, and 8 of those also harboured TERT promoter mutations (OR: 3.65, 95% CI: 0.96–13.90, P =0.06, χ 2 -test; Table 3 ). TERT mRNA expression levels RNA was available from 39 primary melanomas to study relationship between the TERT promoter mutations and gene expression. Of 39 melanomas, 10 carried and 29 did not have the mutations. Of the 10 tumours with the TERT promoter mutations, two harboured −124C>T, one −124/−125CC>TT, two −138/−139CC>TT and five had −146C>T mutations. In addition, RNA was available from five skin tissues from healthy individuals. Analysis of quantitative real-time PCR data showed statistically significant higher levels of mRNA in melanomas with TERT promoter mutations than in tumours without or in skin tissues ( P =0.02, t -test; Fig. 3 ). Figure 3: Relative TERT gene expressions in melanomas with and without TERT promoter mutations. TERT mRNA expression measured by quantitative real-time PCR in skin tissues from healthy individuals ( n =5), tumours without ( n =29) and tumours with the TERT promoter mutations ( n =10). Expression of TERT gene was normalized to GUSB expression, used as an internal standard and quantification was done by ΔΔC T method with log2 transformation. Experiments were carried out in triplicate and box plots represent mean±s.e.m. P values were determined by t -test. Full size image Infinite capability of cancer cells to divide through maintenance of telomeres has been attributed mainly to the sustained expression of telomerase [23] , [24] . Although telomerase is upregulated in over 90% of human cancers, a definite mechanism for its cancer-specific activation has remained unclear [25] , [26] . The detection of the activating somatic mutations in the promoter of the TERT gene has provided an insight into the possible cause of telomerase regeneration [14] . The mutations first detected in melanoma seem to be recurrent in many cancer types [9] , [12] , [15] . In this study we investigated and validated the TERT promoter mutations in a large series of primary melanomas. Within limitations of statistical power, the major findings of the study include the association of the TERT promoter mutations with adverse markers of melanoma prognosis like increased patient age, increased tumour thickness and tumour ulceration. These findings, if confirmed in subsequent studies, coupled with mechanistic relevance of the mutations provide for probable use of the lesions within the TERT promoter in disease management. Earlier in cell lines from metastasized melanoma, we reported a 74% frequency of the somatic TERT promoter mutations and in the same study one-third of primary melanomas were shown to carry those mutations [9] . In this study carried out on 287 primary tumours, we found frequencies of the TERT promoter mutations to be similar to the oncogenic alterations in BRAF . The most frequent TERT promoter mutation in melanoma as described earlier was −146C>T followed by −124C>T (ref. 9 ). In many other cancer types the latter is more frequent than any other TERT promoter mutation [11] , [12] , [27] . Similar to bladder cancer, three melanomas carried the −57A>C as a somatic mutation described initially as a familial melanoma mutation [11] . The underlying discernible selection force behind occurrence of the major TERT promoter mutations is an apparent de novo creation of 5′-CCGGAA/T-3′ binding motif for Ets/TCF transcription factors that leads to an increased gene expression [14] . Abundance of C>T mutations in human cancers in general can be attributed to APOBEC cytidine deaminase expression in cancer development [28] . However, the C>T alterations at the two most recurrent mutational sites in the TERT promoter along with CC>TT tandem mutations at the positions −124/−125 and −138/−139 bp in about 10% of melanomas in this and earlier studies suggested a causal role for ultraviolet exposure in genesis of the lesions. Until now, a CC>TT tandem mutation at the −138/−139 bp positions has been reported in 4 of 1,231 screened bladder cancers compared with 15 of 420 melanomas [29] , [30] . The base change at −139 bp has been reported to be a rare polymorphism represented by rs35550267, the tandem mutation at the position could be caused by a C>T base change at −138 that results in creation of an Ets/TCF-binding motif [9] , [31] . Further support for the association between ultraviolet exposure and TERT promoter mutations was apparent from an increased frequency of the mutations in tumours arising at the sites that are either intermittently or chronically exposed to sunlight compared with rarely exposed parts of the body [32] . Other features that supported the same proposition included association of the mutations in melanomas arising at the site of solar lentigines, the hyper pigmented lesions that are mostly seen in sun-damaged areas of skin [33] . BRAF mutations, in contrast, have been shown to be more prevalent on non-chronically exposed sites than the chronically exposed sites [31] , [32] , [34] . Mutations in melanoma from patients with increased age are considered to be consequences of cumulative exposure to sun. The TERT promoter mutations in contrast to BRAF mutations were more frequent in melanoma from patients with increased age at the diagnosis [32] . Tumour thickness and ulceration in melanoma have persistently been shown to be markers of poor survival and increased risk of death; we found that TERT promoter mutations were associated with both increased Breslow thickness and the presence of tumour ulceration [35] , [36] . The mutations were also associated with vertical growth phase and with the presence of regional and distant metastasis. Histopathological subtypes are now usually considered as biologically distinct entities with the majority being either superficial spreading or NMs [37] . We found that more than half of all NMs compared with one-third of superficial spreading melanomas carried the TERT promoter mutations; tumours with acral lentigous melanoma and lentigo maligna melanoma had fewer mutations. While acral melanomas are characterized by the presence of KIT mutations, BRAF mutations are more frequent in superficial spreading melanoma than NM [34] , [37] . Another distinct feature of NM is the lack of radial growth phase and exclusive progression in vertical manner, which was found to be associated with the presence of the TERT promoter mutations. However, NMs tend to be diagnosed at later stages bearing an increased Breslow thickness, which was reflected in a multivariate model [38] . Beyond the possibility that TERT promoter mutations could be the markers of adverse outcome in melanoma, increased TERT expression as a consequence of the mutations may play a role in tumour growth. Any reduction in the levels of the telomerase across the organisms results in erosion of telomeres. Telomerase reactivation in tumours with telomere dysfunction reportedly leads to malignant progression of prostate cancer in a mouse model [39] . Conversely, suppression of telomerase activity has been shown to significantly reduce tumour invasion and metastatic potential in a melanoma mouse model [40] . The observed effects like induction of dendritic morphology, increased melanin content and tyrosinase expression were reportedly mediated through downregulation of several glycolytic pathway genes [40] . In a subset of tumours where we could measure gene expression, melanomas with the mutations did show an increased TERT transcription compared with melanoma without mutations, in accordance with earlier studies on thyroid tumours, gliomas, malignant pleural mesothelioma and hepatocellular carcinoma [13] , [16] , [17] , [18] . A study on glioma has shown that the TERT promoter mutations rather than hypermethylation are the main mechanism that upregulate the gene expression [14] . Previously, we showed that the TERT promoter mutations tend to be more frequent in tumours with BRAF mutations and in this study we confirmed that association [9] . In a subset of tumours, we also observed co-occurrence of the alterations in TERT promoter and CDKN2A that was higher than what would be expected per chance. Most melanocytic nevi carry BRAF mutations, whereas TERT promoter mutations and CDKN2A alterations are detected in later stages [9] , [41] . The loss of CDKN2A has been suggested to be a key step in escape of melanocytes from BRAF -induced senescence; the acquisition of the TERT promoter mutations and consequent increased telomerase activity can be hypothesized to facilitate stabilization of the transformed genome following telomeric crisis through reversal of telomeric loss as a consequence of increase telomerase activity [42] , [43] . Thus, alterations in BRAF or NRAS , CDKN2A and TERT promoter can be presumed to represent unique driver mutations en route to melanoma development. The TERT promoter mutations represent novel genetic alterations with a role in cancer development through alteration in gene expression. In this study based on a relatively large series of primary melanoma, we showed association of the TERT promoter mutations with factors that are generally considered as markers of poor prognosis. Owing to limited numbers of events in the set of patients included in this study, we could not determine whether the mutations influence melanoma-specific survival or recurrence. Strategies based on therapeutic inhibition of telomerase that include small molecular inhibitors, immunotherapy, gene therapy, telomere and telomerase proteins are already part of clinical trials [44] . Further research will determine usefulness of the TERT promoter mutations in the context of melanoma treatment where strategies based on BRAF inhibitors have shown a vast potential despite persistent issue of resistance [45] . Patients and tumour samples In this study, primary tumours from 287 melanoma patients diagnosed between October 2000 and December 2012 were retrieved from the biobank of the Instituto Valenciano de Oncología in Valencia, Spain. The patients included in the study were being treated at the same institute during that period. Of 287 patients, 213 presented only localized disease (stages I and II), 74 had also developed locoregional (stage III) and 4 had also presented distant disease (stage IV). Sixty tumours were fresh frozen and 227 were available as FFPE tissue. From six patients, corresponding metastases were also available as FFPE. For fresh frozen tumours, tissues were excised from part of skin with clinically and dermoscopically confirmed melanoma. Excised tissues were divided into two parts, one part was immediately frozen in liquid nitrogen and the second part was investigated by a pathologist to check the presence of tumour cells. Only tissues with 70% or more tumour cells were included in the investigation. All patient data were obtained from the melanoma database of the institution. The database, initiated in January 2000, contains systematically and prospectively collected information from patients treated at the institution [46] . Ethical approval for the study from the institutional review board of the Instituto Valenciano de Oncología and written informed consent from all study patients were obtained. Phenotypic characteristics and sun exposure history Details on collection of clinical, epidemiological and histological data have been described previously [46] . In brief, patients underwent clinical examination by expert dermatologists in which congenital, atypical and common melanocytic nevi (>2 mm in diameter) were counted. The presence or absence of actinic keratoses and solar lentigines was also recorded. The density of freckling in childhood on the face, arm and back was scored according to the Vancouver charts [47] . Patients were also asked to report their sun exposure history recording the total number of severe and light sunburns. Hair and eye colour, as well as the skin type using the Fitzpatrick classification was also recorded. Family and personal histories of other neoplasia were systematically collected. The pattern of sun exposure was inferred from medical histories, physical examinations, patient reported data and the location of the primary tumour, and was assigned into three categories, rarely exposed, usually exposed and infrequently exposed. The assumptions about sun exposure based only on melanoma site were avoided [46] . MC1R genotype data were obtained by direct sequencing of available constitutional DNA from the patients included in the study and had been deposited in biobank [48] . DNA and RNA extraction From fresh frozen melanoma samples, DNA and RNA were extracted using the QIAGEN AllPrep DNA/RNA MiniKit. Tissues were homogenized in a Tissuelyser LT (Qiagen, Hilden, Germany) with 5 mm stainless steel beads in 600 μl RLT buffer and were further processed. Concentrations of total DNA and RNA were measured using an ultraviolet–visible spectrophotometer (NanoDrop Technologies, Wilmington, USA) and absorption ratio at 260/280 nm was determined. RNA consistency was examined on a Bioanalyzer 2100 System (Agilent Technologies, Palo Alto, CA) using the corresponding RNA nanochips. For extraction of DNA from FFPE melanoma tissue following method was used. Haematoxylin and eosin-stained sections of FFPE tissues were examined for tumour content by a pathologist. Neoplastic areas were selected and dissected by tru-cut (2−3 × 0.6 μm) from the paraffin blocks with a manual tissue arrayer (Breecher MTA-I) to avoid stromal cells and to increase the specificity of melanoma cells more than 95%. DNA was isolated using Qiagen DNeasy Tissue Kit (Qiagen) with additional proteinase K digestion at 55 °C for 48 h (ref. 49 ). Mutations in different genes Mutational status of the TERT core promoter region (from position −27 to −286 from ATG start site) was determined by PCR and Sanger sequencing. PCR was carried out in a 10-μl volume containing 10 ng DNA, 50 mM KCl, 0.11 mM dNTP and 0.11 μM of each primer. Concentrations of MgCl 2 and other additives and temperature conditions were adjusted according to the primer sequences ( Supplementary Table 2 ). Amplified products were purified with Exosap (GE Healthcare, Buckinghamshire, UK) to remove unused primer and were subjected to 35 cycles of sequencing reaction with a dideoxy terminator kit and forward and reverse primers in separate reactions (BigDyeTerminator v3.1 Cycle Sequencing Kit, Applied Biosystems, Austin, TX, USA). Sequencing reaction products were precipitated with ethanol and analysed on a capillary sequencer (AbiPrism 3130xl Genetic Analyzer). Mutations at codon 600 of BRAF p.V600 and codon 61 of NRAS p.Q61 in DNA from FFPE samples were detected with single base extension or allele-specific assays using the iPLEX genotyping format (Sequenom) [49] . For DNA from fresh frozen tumour tissues, PCR and Sanger sequencing as described were used to detect mutations in the TERT promoter, BRAF , NRAS and additionally in CDKN2A . Thirteen FFPE samples with known BRAF status were re-sequenced with Sanger sequencing for random confirmation of the results. The sequencing data were analysed using Geneious Pro 5.6.5 software with reference to the sequences from the NCBI gene database, TERT (chr5: 1,295,071–1,295,521), BRAF (NG_007873.2), NRAS (NG_007572.1) and CDKN2A (NC_000009.11; NM_000077.4). CDKN2A deletion and methylation screening by MS-MLPA To detect deletions and methylation at the CDKN2A locus, we used the MS-MLPA method with specific probes (SALSA MLPA ME024 9p21 CDKN2A /2B; MRC Holland, Amsterdam, The Netherlands). Fifty nanograms of DNA per sample was subjected to 16 h of incubation with the probe mix and afterwards divided into two reactions. One was processed in a ligation reaction, followed by a multiplex PCR. The second part was processed in a ligation step followed by Hha I digestion and then amplified in a multiplex PCR. Fragment analysis was performed on a capillary sequencer (AbiPrism 3130xl Genetic Analyzer). The results were evaluated using Coffalyser software (MRC Holland); threshold to define deletions was set at the delta value of 0.3 and if methylation of a probe exceeded 30% the status was considered positive. Measurement of the TERT gene expression For measurement of the TERT expression, reverse transcription reaction was performed using between 0.75 and 1.0 μg RNA and random hexamer primers using a cDNA synthesis kit (Thermo Scientific, Waltham, USA). TERT expression levels were then determined by quantitative real-time PCR using a Syber Green kit (Qiagen). The real-time PCR was carried out in triplicates on a 384-well layout using forward (5′-CGGAAGAGTGTCTGGAGCAA-3′; biding site in exon 3 of TERT ) and reverse (5′-GGATGAAGCGGAGTCTGGA-3′; binding site in exon 4 of TERT ) primers specific for TERT and primers for the GUSB gene (Qiagen), a housekeeping gene used as an internal standard. TERT expression levels were calculated using GUSB expression as a reference and relative quantification was performed using the ΔΔ C T method and log2 transformation. Statistical analysis The associations between the TERT promoter mutations and other parameters were determined by χ 2 -test. A difference was considered statistically significant if P value was<0.05. ORs were calculated to assess the size of the effect of different parameters on the occurrence of the TERT promoter mutations. Multivariate logistic regression was also carried out that included age at diagnosis, histological type, presence of solar lentigines and pattern of sun exposure at melanoma site, ulceration, stage and Breslow thickness that were associated with the mutations in the univariate analyses. How to cite this article: Heidenreich, B. et al. Telomerase reverse transcriptase promoter mutations in primary cutaneous melanoma. Nat. Commun. 5:3401 doi: 10.1038/ncomms4401 (2014).